KCNQ5 K+channels control hippocampal synaptic inhibition and fast network oscillations KCNQ2 (Kv7.2) and KCNQ3 (Kv7.3) K + channels dampen neuronal excitability and their functional impairment may lead to epilepsy. Less is known about KCNQ5 (Kv7.5), which also displays wide expression in the brain. Here we show an unexpected role of KCNQ5 in dampening synaptic inhibition and shaping network synchronization in the hippocampus. KCNQ5 localizes to the postsynaptic site of inhibitory synapses on pyramidal cells and in interneurons. Kcnq5 dn/dn mice lacking functional KCNQ5 channels display increased excitability of different classes of interneurons, enhanced phasic and tonic inhibition, and decreased electrical shunting of inhibitory postsynaptic currents. In vivo , loss of KCNQ5 function leads to reduced fast (gamma and ripple) hippocampal oscillations, altered gamma-rhythmic discharge of pyramidal cells and impaired spatial representations. Our work demonstrates that KCNQ5 controls excitability and function of hippocampal networks through modulation of synaptic inhibition. K CNQ genes encode five voltage-gated potassium channels in mammals (KCNQ1–5 or K v 7.1–K v 7.5) and mutations in KCNQ1 – 4 underlie human diseases [1] , [2] . KCNQ1 mutations entail cardiac arrhythmias and deafness, mutations in KCNQ2 and -3 lead to benign familial neonatal convulsions [3] , [4] , [5] and KCNQ4 mutations can cause progressive hearing loss [6] . KCNQ5 has not yet been linked directly to human disease, although KCNQ5 is deleted together with other genes in some patients with mental retardation [7] , [8] and dysfunction of KCNQ3/KCNQ5 heteromers has been associated with autism disorders [9] . In the brain, KCNQ subunits 2, -3 and -5 show wide neuronal expression, whereas KCNQ4 is restricted to specific brain stem nuclei including parts of the auditory pathway [10] . KCNQ4 is also found in the inner ear [6] and a subset of touch receptors in the skin [11] . KCNQ2 and -3 localize to axon initial segments and nodes of Ranvier [12] , [13] . KCNQ2/KCNQ3 heteromers are considered to be a molecular correlate of the M-current [14] , [15] . These currents are partially active at resting membrane potential and their inhibition by G-protein-coupled receptors increases neuronal excitability. In addition, KCNQ2 and -3 mediate components of the medium and slow afterhyperpolarization (AHP) currents in hippocampal neurons [16] , [17] , [18] . Compared with KCNQ2, -3 and -4, little is known about the function of KCNQ5. KCNQ5 is widely expressed throughout the brain [13] , [19] , [20] . In the hippocampus, KCNQ5 contributes to AHP currents in the CA3 area [13] . KCNQ5 was reported to localize mainly to neuronal cell somata and dendrites in human cortex and hippocampus [21] , to glutamatergic synapses in several rat brain stem nuclei [22] , [23] and to the postsynaptic membrane of vestibular calyx terminals [24] . Furthermore, KCNQ5 was proposed to be located at the presynaptic membrane of the calyx of Held and to control its properties [23] . Here we show that in the mouse hippocampus, where it is most highly expressed in the CA3 area, KCNQ5 localizes to both pyramidal cells and all investigated subtypes of inhibitory interneurons. Immunolabelling reveals KCNQ5 clustering at postsynaptic membranes of GABAergic synapses. To elucidate the global physiological function of KCNQ5, we used Kcnq5 dn/dn mice that carry a dominant negative mutation (G278S) in the pore loop [13] , resulting in a non-conducting mutant protein. This functional ablation of KCNQ5 results in alterations of synaptic inhibition and excitability in the hippocampus in vitro and in vivo . Fast network oscillations, gamma-rhythmic firing of pyramidal cells and spatial representations are impaired in freely moving Kcnq5 dn/dn mice. Our work shows that KCNQ5 modulates hippocampal synaptic inhibition and network synchrony and unveils an important role of KCNQ5 in hippocampal information processing. KCNQ5 expression in pyramidal cells and interneurons KCNQ5 is widely expressed in many brain regions [19] , [20] . In the hippocampus, mRNA hybridization (Allen brain atlas, http://www.brain-map.org/ ) and immunohistochemistry revealed higher KCNQ5 expression in the CA3 than CA1 hippocampal region [13] . Immunolabelling with our KCNQ5 antibody was intense in strata oriens and radiatum, regions that harbour extensive synaptic contacts ( Fig. 1a ). In CA3, there was a gradient of KCNQ5 expression from CA3a (close to CA2) towards the CA3c area (close to dentate gyrus). In the absence of mice lacking KCNQ5 expression, the specificity of KCNQ5 labelling was confirmed with Kcnq5 dn/dn knock-in mice [13] , which express a dominant-negative (dn), non-conducting pore mutant (G278S) of KCNQ5 (ref. 20 ). In these mice, the pattern of KCNQ5 labelling of the hippocampus was changed ( Fig. 1b ). Labelling was reduced in the CA1 area, suggesting that the mutant protein might be less stable. In CA3, KCNQ5 immunoreactivity was shifted from the stratum (st.) radiatum and st. oriens to pyramidal cell bodies ( Fig. 1b,c ). 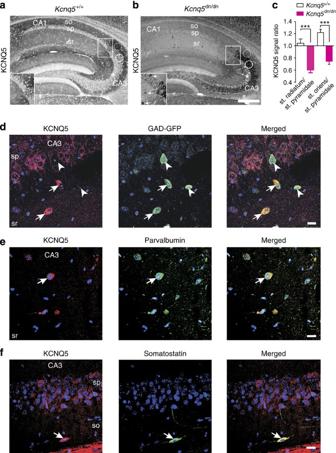Figure 1: Hippocampal expression of KCNQ5 in WT andKcnq5dn/dnmice. (a) Dark immunostaining showed KCNQ5 expression in the hippocampus, which is particularly strong in the CA3 area. (b) Altered expression of the mutant KCNQ5G278Sprotein in hippocampus ofKcnq5dn/dnmice. Insets inaandbshow higher magnification. Arrows inbshow labelled cells outside the pyramidal cell layer. Scale bar inbfor (a,b): 0.25 cm. Asterisk: st. lucidum in the CA3 area. (c) Inverted ratio of KCNQ5 labelling (mean±s.e.m.) in st. pyramidale (solid white circle ina,b), st. radiatum (dotted black circle ina,b) and st. oriens (dotted white circle ina,b) in hippocampi ofKcnq5dn/dnmice. WT: 8 hippocampi;Kcnq5dn/dn: 6 hippocampi, ***P<0.0001 (Student’st-test). (d–f) KCNQ5 expression in CA3 interneurons ofKcnq5dn/dnmice. (d) Hippocampi ofKcnq5dn/dn× GAD-GFP mice were labelled with KCNQ5 (red) and GFP (green) antibodies. A subset of GAD-GFP-positive interneurons in CA3 st. radiatum was co-labelled for KCNQ5 (arrows). Arrowheads, GFP-positive interneurons not labelled for KCNQ5. Scale bar, 20 μm. sp: st. pyramidale; sr: st. radiatum. (e) Co-labelling of a st. radiatum parvalbumin-positive interneuron with KCNQ5, and (f) of a st. oriens somatostatin-positive interneuron with KCNQ5 antibody. Co-labelled cells highlighted by arrows. For other interneuron markers and statistics, seeSupplementary Fig. 2. Scale bars, 20 μm. Figure 1: Hippocampal expression of KCNQ5 in WT and Kcnq5 dn/dn mice. ( a ) Dark immunostaining showed KCNQ5 expression in the hippocampus, which is particularly strong in the CA3 area. ( b ) Altered expression of the mutant KCNQ5 G278S protein in hippocampus of Kcnq5 dn/dn mice. Insets in a and b show higher magnification. Arrows in b show labelled cells outside the pyramidal cell layer. Scale bar in b for ( a , b ): 0.25 cm. Asterisk: st. lucidum in the CA3 area. ( c ) Inverted ratio of KCNQ5 labelling (mean±s.e.m.) in st. pyramidale (solid white circle in a , b ), st. radiatum (dotted black circle in a , b ) and st. oriens (dotted white circle in a , b ) in hippocampi of Kcnq5 dn/dn mice. WT: 8 hippocampi; Kcnq5 dn/dn : 6 hippocampi, *** P <0.0001 (Student’s t -test). ( d – f ) KCNQ5 expression in CA3 interneurons of Kcnq5 dn/dn mice. ( d ) Hippocampi of Kcnq5 dn/dn × GAD-GFP mice were labelled with KCNQ5 (red) and GFP (green) antibodies. A subset of GAD-GFP-positive interneurons in CA3 st. radiatum was co-labelled for KCNQ5 (arrows). Arrowheads, GFP-positive interneurons not labelled for KCNQ5. Scale bar, 20 μm. sp: st. pyramidale; sr: st. radiatum. ( e ) Co-labelling of a st. radiatum parvalbumin-positive interneuron with KCNQ5, and ( f ) of a st. oriens somatostatin-positive interneuron with KCNQ5 antibody. Co-labelled cells highlighted by arrows. For other interneuron markers and statistics, see Supplementary Fig. 2 . Scale bars, 20 μm. Full size image We neither detected compensatory changes in the expression of other KCNQ family members [13] or of several Kir K + channels ( Supplementary Fig. 1a ). The overall normal brain histomorphology of Kcnq5 dn/dn mice [13] and the unchanged expression of several synaptic proteins in these mice ( Supplementary Fig. 1b ) further suggested that the reduced KCNQ5 labelling of st. radiatum and oriens is not owed to neurodegeneration. As KCNQ4 channels with an equivalent pore mutation (G285S) [6] show diminished plasma membrane localization in heterologous expression systems [25] and in vivo [11] , [24] , we rather suspected abnormal protein trafficking as the underlying cause. Indeed, when expressed in Xenopus oocytes, KCNQ5 G278S subunits carrying an extracellular HA-tag displayed reduced plasma membrane localization compared with similarly tagged wild-type (WT) KCNQ5 ( Supplementary Fig. 1c,d ). This effect was observed either when KCNQ5 G278S was expressed alone or together with KCNQ3, which can form heteromers with KCNQ5 (refs 19 , 20 ). Hence, the altered staining pattern of Kcnq5 dn/dn hippocampi likely resulted from impaired trafficking of the mutant non-conducting protein. Instead of reaching their normal peripheral position on neurites, KCNQ5 G278S mutant channels remain in somata of pyramidal cells, similar to the recently described retention of this mutant in somata of vestibular ganglion cells [24] . In addition to confirming the specificity of our immunolabelling experiments, the trafficking defect of the KCNQ5 G278S mutant facilitated the identification of cell types expressing KCNQ5. The shift of immunoreactivity from st. oriens and st. radiatum to pyramidal cell somata ( Fig. 1a–c ) indicated that a sizeable portion of KCNQ5 is present on neurites of pyramidal cells. In Kcnq5 dn/dn , but not in Kcnq5 +/+ hippocampi, immunostaining revealed KCNQ5-positive cell somata also outside of the pyramidal layer, for example, in the st. radiatum ( Fig. 1b ). This preferential labelling of Kcnq5 dn/dn somata likely results from a retention of the mutant protein in cell bodies, where, in contrast to the WT situation, it can be distinguished from diffuse background labelling. Indeed, in situ hybridization revealed similar labelling outside the pyramidal cell layer in Kcnq5 +/+ and Kcnq5 dn/dn mice ( Supplementary Fig. 2a,b ). To examine whether these cells corresponded to inhibitory interneurons, we crossed Kcnq5 dn/dn mice to GAD67-GFP mice that specifically label GABAergic neurons [26] ( Fig. 1d ). Indeed, 12.3% (98/781 cells from three mice) of GFP-positive cells in Kcnq5 dn/dn × GAD67-GFP +/− mice were robustly labelled for KCNQ5. KCNQ5-labelled interneurons were found in the st. radiatum, oriens and lacunosum-moleculare ( Fig. 1b,d–f ). The KCNQ5 signal in Kcnq5 dn/dn mice overlapped with markers for various types of interneurons like parvalbumin and somatostatin ( Fig. 1e,f ) and calretinin and neuropeptide Y ( Supplementary Fig. 3a–c ). A sizeable fraction of interneurons stained with any of the interneuron markers was unambiguously labelled for KCNQ5 ( Supplementary Fig. 3d ). Likewise, combining in situ hybridization with immunohistochemistry, parvalbumin- and somatostatin-positive interneurons were found to express Kcnq5 mRNA in both Kcnq5 +/+ and Kcnq5 dn/dn hippocampi ( Supplementary Fig. 2c–f ). Hence, in addition to hippocampal pyramidal cells, KCNQ5 is widely expressed in hippocampal interneurons of different subtypes. Increased excitability of Kcnq5 dn/dn interneurons The KCNQ5 G278S mutant does not yield K + -currents by itself and exerts dominant-negative effects on co-expressed KCNQ3, -4 and -5 subunits [13] , [20] , [24] . Kcnq5 dn/dn mice, which carry the G278S mutation on both alleles, are therefore expected to lack currents from homo- or heteromeric channels carrying at least one KCNQ5 subunit. By contrast, the consequences of a deletion of KCNQ5 in Kcnq5 −/− mice are difficult to predict. In some cells, the number of KCNQ2/KCNQ3 channels may increase because KCNQ5 no longer competes with KCNQ2 for KCNQ3 binding. As KCNQ2/KCNQ3 heteromers yield large K + -currents [27] , Kcnq5 −/− mice may display phenotypes resulting from both a decrease and increase of specific K + currents. Our approach, that is, the use of Kcnq5 dn/dn mice avoids all these complications and allowed us to specifically investigate the role of KCNQ5 in hippocampal slices and in vivo . The identification of KCNQ5 in interneurons prompted us to investigate intrinsic excitability of interneurons in the CA3 after blocking synaptic transmission. To identify interneurons, we crossed Kcnq5 dn/dn mice with mice expressing GFP under control of the GAD67 promotor. Recorded cells were filled with biocytin by the patch pipette and 59 cells could be subsequently classified morphologically into basket, bistratified and oriens-lacunosum-moleculare interneurons. All three types of interneuron ( Fig. 2a–c ) displayed increased excitability in Kcnq5 dn/dn mice as indicated by a larger number of action potentials in response to depolarizing current injections ( Fig. 2d–i ). We likewise observed an increased excitability in non-classified interneurons in st. radiatum ( Supplementary Fig. 4a ). In contrast to interneurons, the excitability of CA3 and CA1 pyramidal cells appeared unchanged ( Supplementary Fig. 4b,c ). Resting membrane potential was not altered in either cell type ( Supplementary Fig. 4d,e ). 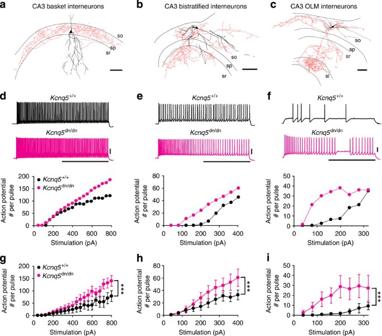Figure 2: Excitability ofKcnq5dn/dninterneurons in the CA3 area. (a–c) Camera lucida reconstructions of three distinct subpopulations of interneurons identified bypost-hoclabelling: somatic targeting CA3 basket cells (a), dendritic targeting CA3 bistratified cells (b) and dendritic targeting CA3 OLM (oriens-lacunosum-moleculare) cells (c). Dendrites and cell bodies in black, axons in red. so, st. oriens; sp, st. pyramidale; sr, st. radiatum. Scale bars, 100 μm. (d–f) Example responses to a depolarizing current pulse (1 s) from each subpopulation of interneurons shown as voltage traces (basket cells (d): 600 pA; bistratified cells (e): 440 pA; OLM cells (f): 160 pA) and number of action potentials plotted against injected current. Scale bars, 20 mV, 500 ms. (g–i) Number of action potentials per pulse (mean±s.e.m.) plotted against injected current for all investigated cells (basket cells (g): WT: 7 cells, 4 mice;Kcnq5dn/dn: 13 cells, 9 mice; bistratified cells (h): WT: 15 cells, 10 mice;Kcnq5dn/dn: 9 cells, 4 mice; OLM cells (i): WT: 7 cells, 5 mice;Kcnq5dn/dn: 8 cells, 4 mice). ***P<0.001 (analysis of variance). Figure 2: Excitability of Kcnq5 dn/dn interneurons in the CA3 area. ( a – c ) Camera lucida reconstructions of three distinct subpopulations of interneurons identified by post-hoc labelling: somatic targeting CA3 basket cells ( a ), dendritic targeting CA3 bistratified cells ( b ) and dendritic targeting CA3 OLM (oriens-lacunosum-moleculare) cells ( c ). Dendrites and cell bodies in black, axons in red. so, st. oriens; sp, st. pyramidale; sr, st. radiatum. Scale bars, 100 μm. ( d – f ) Example responses to a depolarizing current pulse (1 s) from each subpopulation of interneurons shown as voltage traces (basket cells ( d ): 600 pA; bistratified cells ( e ): 440 pA; OLM cells ( f ): 160 pA) and number of action potentials plotted against injected current. Scale bars, 20 mV, 500 ms. ( g – i ) Number of action potentials per pulse (mean±s.e.m.) plotted against injected current for all investigated cells (basket cells ( g ): WT: 7 cells, 4 mice; Kcnq5 dn/dn : 13 cells, 9 mice; bistratified cells ( h ): WT: 15 cells, 10 mice; Kcnq5 dn/dn : 9 cells, 4 mice; OLM cells ( i ): WT: 7 cells, 5 mice; Kcnq5 dn/dn : 8 cells, 4 mice). *** P <0.001 (analysis of variance). Full size image Enhanced hippocampal GABAergic inhibition in Kcnq5 dn/dn mice The increased excitability of interneurons suggested that the functional loss of KCNQ5 would boost synaptic inhibition in the CA3 area. Indeed, we observed an increase in the frequency of spontaneous inhibitory postsynaptic currents (sIPSCs) in Kcnq5 dn/dn CA3 pyramidal cells and a shift of their mean amplitudes to larger values ( Fig. 3a–d ). By contrast, neither frequency nor amplitude of spontaneous excitatory postsynaptic currents (sEPSCs) were altered in Kcnq5 dn/dn CA3 pyramidal cells ( Supplementary Fig. 4f ). Moreover, inhibition of extrasynaptic GABA A receptors in voltage-clamp experiments suggested that ambient GABA (γ-aminobutyric acid) was increased in Kcnq5 dn/dn CA3 pyramidal cells ( Supplementary Fig. 4g,h ). Because KCNQ channels can be inhibited by muscarinic M1 receptors [14] , [28] and since hippocampal circuits are modulated by cholinergic input [29] , [30] , we tested the effect of the muscarinic agonist carbachol. Transient application of carbachol (20 μM) markedly increased both sIPSC amplitude and frequency in WT CA3 pyramidal cells ( Fig. 3a–d ). This effect was absent in Kcnq5 dn/dn slices, indicating a major contribution of KCNQ5 to acetylcholine-mediated control of inhibition in CA3. In addition to sIPSCs, we also investigated effects on inhibitory postsynaptic currents (IPSCs) of pyramidal cells that were evoked by extracellular stimulation in st. radiatum close to the recorded cell. Consistent with our results on sIPSCs, also evoked IPSCs were significantly larger in Kcnq5 dn/dn mice compared with controls ( Fig. 3e ). 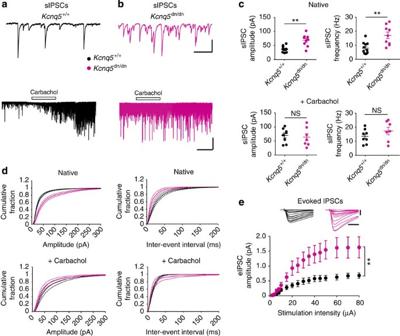Figure 3: Enhanced inhibition in the CA3 area ofKcnq5dn/dnmice. (a–c) GABAergic synaptic transmission in the CA3 area. Example traces of spontaneous IPSC (sIPSC) recorded in CA3 pyramidal cells from WT (a, black) andKcnq5dn/dn(b, red) mice under control conditions (top) and upon short application of the muscarinic agonist carbachol (bottom). Scale bars, 200 pA, 400 ms (top) and 20 s (bottom). (c) Summary of changes in frequency and amplitude of individual recordings. Mean values and s.e.m. indicated by lines. Top: WT: 11 cells, 4 mice;Kcnq5dn/dn: 9 cells, 4 mice,P<0.01. Bottom: WT: 8 cells, 4 mice;Kcnq5dn/dn: 7 cells, 4 mice. **P<0.01 (Student’st-test). (d) Cumulative distribution plots for data shown inc. (e) Evoked IPSCs (mean±s.e.m.) in CA3 pyramidal cells from WT (8 cells, 4 mice) andKcnq5dn/dnmice (9 cells, 4 mice). **P<0.01 (analysis of variance). Input/output curves (IPSC amplitudes as function of stimulus intensity) and example traces of evoked IPSCs in CA3 pyramidal cells. IPSCs were recorded in the absence of glutamatergic transmission (blocked by CNQX/AP5 in bath) and were evoked by a stimulation electrode placed nearby in the st. radiatum. Scale bars, 500 pA, 25 ms. Figure 3: Enhanced inhibition in the CA3 area of Kcnq5 dn/dn mice. ( a – c ) GABAergic synaptic transmission in the CA3 area. Example traces of spontaneous IPSC (sIPSC) recorded in CA3 pyramidal cells from WT ( a , black) and Kcnq5 dn/dn ( b , red) mice under control conditions (top) and upon short application of the muscarinic agonist carbachol (bottom). Scale bars, 200 pA, 400 ms (top) and 20 s (bottom). ( c ) Summary of changes in frequency and amplitude of individual recordings. Mean values and s.e.m. indicated by lines. Top: WT: 11 cells, 4 mice; Kcnq5 dn/dn : 9 cells, 4 mice, P <0.01. Bottom: WT: 8 cells, 4 mice; Kcnq5 dn/dn : 7 cells, 4 mice. ** P <0.01 (Student’s t -test). ( d ) Cumulative distribution plots for data shown in c . ( e ) Evoked IPSCs (mean±s.e.m.) in CA3 pyramidal cells from WT (8 cells, 4 mice) and Kcnq5 dn/dn mice (9 cells, 4 mice). ** P <0.01 (analysis of variance). Input/output curves (IPSC amplitudes as function of stimulus intensity) and example traces of evoked IPSCs in CA3 pyramidal cells. IPSCs were recorded in the absence of glutamatergic transmission (blocked by CNQX/AP5 in bath) and were evoked by a stimulation electrode placed nearby in the st. radiatum. Scale bars, 500 pA, 25 ms. Full size image KCNQ5 localizes to inhibitory synapses As KCNQ5 was expressed in layers rich in synaptic contacts ( Fig. 1a ), we asked whether this protein might be found at synapses. Indeed, KCNQ5 co-localized with gephyrin ( Fig. 4a,f ), a postsynaptic marker for GABAergic and glycinergic synapses, and partially overlapped with presynaptic markers like the vesicular GABA transporter vGAT and the GABA-synthesizing enzyme GAD65/67 ( Fig. 4b,c ). Co-localization with markers for inhibitory synapses was not only seen in st. oriens or radiatum, but also on pyramidal cell bodies that were decorated by KCNQ5-positive puncta ( Fig. 4c ). Most gephyrin-positive CA3 synapses were KCNQ5-positive (64.3±2.3% and 82.5±1.7% in st. oriens and radiatum, respectively). Vice-versa, 66.5±3% and 63.4±3.9% of KCNQ5-positive dots in the CA3 st. oriens and st. radiatum, respectively, were co-labelled with gephyrin (748 and 641 synapses, respectively, from three mice). KCNQ5 localized to inhibitory synapses also in other brain regions like the cerebellum (not shown) and the brainstem ( Supplementary Fig. 5a,b ). KCNQ5 was not found at glutamatergic terminals that were labelled for the glutamate receptor subunit GluR2 or the vesicular glutamate transporter vGlut1 ( Fig. 4d,e ). As described previously [22] , [23] , KCNQ5 immunoreactivity was found at calyces of Held ( Supplementary Fig. 5a,b ). Closer examination, however, revealed that KCNQ5 did not co-localize with vGlut1 at the presynaptic membrane ( Supplementary Fig. 5a ), but rather with gephyrin ( Supplementary Fig. 5b ) that marks inhibitory synapses, which contact this giant excitatory synaptic bouton [31] . 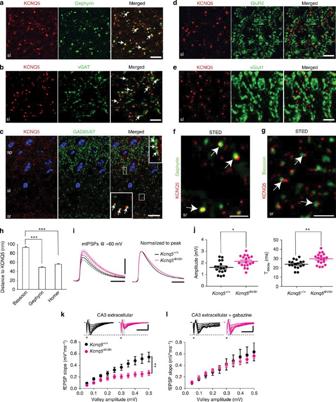Figure 4: KCNQ5 localizes to inhibitory synapses. (a–g) KCNQ5 localization in the CA3 area. Sections were labelled for KCNQ5 (a–g, red), gephyrin (a,fgreen), vGAT (b, green), GAD65/67 (c, green), GluR2 (d, green), vGlut1 (e, green) and bassoon (g, green) antibodies. Boxed areas in (c): inhibitory synapses on pyramidal cell bodies (top right) and in st. radiatum (bottom left). (f,g) STED microscopy of CA3 sections. KCNQ5 co-localizes with postsynaptic gephyrin (f), but not with presynaptic bassoon (g). (h) Mean distances (± s.e.m.) between KCNQ5 and bassoon, gephyrin, and homer from 240 CA3 synapses/pair. ***P<0.001 (analysis of variance (ANOVA)). Scale bars: for (a,b,d,e), 10 μm; for (c), 20 μm; for (f,g), 1 μm. sp: st. pyramidale; sl: st. lucidum; sr: st. radiatum. Arrows, co-localization of KCNQ5 with inhibitory synapse markers. (i,j) Miniature inhibitory postsynaptic potentials (mIPSPs) from WT (black, 17 cells, 4 mice) andKcnq5dn/dnmice (red, 18 cells, 4 mice). (i) Left, averaged time courses of mIPSPs (solid lines) and 95% confidence intervals (dotted lines). Right, normalized mIPSPs reveal slower decay kinetics inKcnq5dn/dnthan in WT mice. (j) mIPSP amplitudes and decay times for each recorded cell. Means and s.e.m. indicated by lines. *P<0.05, **P<0.01 (Student’st-test). Scale bars, 1 mV, 20 ms. (k,l) Extracellular field potentials (fEPSPs) recorded in st. radiatum of CA3 in hippocampal slices from WT (black) andKcnq5dn/dn(red) mice in CA3 in the absence (k, WT: 12 slices, 5 mice;Kcnq5dn/dn: 13 slices, 5 mice, **P<0.01, ANOVA) and presence (l, WT: 8 slices, 3 mice;Kcnq5dn/dn: 8 slices, 3 mice, not significant (NS)) of gabazine. Presynaptic volleys and fEPSP slopes highlighted in traces by asterisks and rectangles, respectively. Scale bars, 0.25 mV, 10 ms. Figure 4: KCNQ5 localizes to inhibitory synapses. ( a – g ) KCNQ5 localization in the CA3 area. Sections were labelled for KCNQ5 ( a – g , red), gephyrin ( a , f green), vGAT ( b , green), GAD65/67 ( c , green), GluR2 ( d , green), vGlut1 ( e , green) and bassoon ( g , green) antibodies. Boxed areas in ( c ): inhibitory synapses on pyramidal cell bodies (top right) and in st. radiatum (bottom left). ( f , g ) STED microscopy of CA3 sections. KCNQ5 co-localizes with postsynaptic gephyrin ( f ), but not with presynaptic bassoon ( g ). ( h ) Mean distances (± s.e.m.) between KCNQ5 and bassoon, gephyrin, and homer from 240 CA3 synapses/pair. *** P <0.001 (analysis of variance (ANOVA)). Scale bars: for ( a , b , d , e ), 10 μm; for ( c ), 20 μm; for ( f , g ), 1 μm. sp: st. pyramidale; sl: st. lucidum; sr: st. radiatum. Arrows, co-localization of KCNQ5 with inhibitory synapse markers. ( i , j ) Miniature inhibitory postsynaptic potentials (mIPSPs) from WT (black, 17 cells, 4 mice) and Kcnq5 dn/dn mice (red, 18 cells, 4 mice). ( i ) Left, averaged time courses of mIPSPs (solid lines) and 95% confidence intervals (dotted lines). Right, normalized mIPSPs reveal slower decay kinetics in Kcnq5 dn/dn than in WT mice. ( j ) mIPSP amplitudes and decay times for each recorded cell. Means and s.e.m. indicated by lines. * P <0.05, ** P <0.01 (Student’s t -test). Scale bars, 1 mV, 20 ms. ( k , l ) Extracellular field potentials (fEPSPs) recorded in st. radiatum of CA3 in hippocampal slices from WT (black) and Kcnq5 dn/dn (red) mice in CA3 in the absence ( k , WT: 12 slices, 5 mice; Kcnq5 dn/dn : 13 slices, 5 mice, ** P <0.01, ANOVA) and presence ( l , WT: 8 slices, 3 mice; Kcnq5 dn/dn : 8 slices, 3 mice, not significant (NS)) of gabazine. Presynaptic volleys and fEPSP slopes highlighted in traces by asterisks and rectangles, respectively. Scale bars, 0.25 mV, 10 ms. Full size image High-resolution stimulated emission depletion (STED) microscopy of CA3 synapses showed that KCNQ5 labelling overlapped with postsynaptic gephyrin, but not with presynaptic bassoon ( Fig. 4f,g ). Evaluation of over 200 synapses for each pair revealed a significantly shorter distance of KCNQ5 to the postsynaptic markers gephyrin and homer than to presynaptic bassoon ( Fig. 4h ). Subcellular fractionation ( Supplementary Fig. 5c ) showed the presence of KCNQ5 in the postsynaptic density fractions (PSD) I and II, further supporting a postsynaptic localization. The reduction of KCNQ5 levels in synaptic fractions from Kcnq5 dn/dn relative to WT mice, which exceeded the reduction in total brain homogenate ( Supplementary Fig. 5c ), agreed with the shift of the KCNQ5 G278S mutant from synaptic regions to cell bodies ( Fig. 1a–c ). The overall reduction of KCNQ5 in Kcnq5 dn/dn brain ( Supplementary Fig. 5c ) suggested an increased degradation of the mutant protein and agreed with the reduced KCNQ5 labelling in the CA1 area of Kcnq5 dn/dn mice ( Fig. 1b ). Unlike KCNQ5, KCNQ3 (and KCNQ2, not shown) did not co-localize with synaptic markers ( Supplementary Fig. 6a–c ). As described previously [12] , [13] , [32] , we rather detected these channels at axon initial segments and nodes of Ranvier ( Supplementary Fig. 6d ). Synaptic transmission in Kcnq5 dn/dn hippocampal slices The postsynaptic localization of KCNQ5 ( Fig. 4a–c,f,g ) suggested that it might shunt postsynaptic currents. To check for this possibility, we recorded miniature inhibitory postsynaptic potentials (mIPSPs; current-clamp configuration, ~−60 mV) from CA3 principal neurons and indeed found that both amplitudes and time constants were increased in Kcnq5 dn/dn mice ( Fig. 4i,j and Supplementary Fig. 7b ). In control experiments performed at ~−90 mV, a voltage at which KCNQ5 channels are closed [33] , mIPSPs were comparable in WT and Kcnq5 dn/dn mice ( Supplementary Fig. 7c,d ) supporting our hypothesis of KCNQ5 involvement in shunting. In voltage-clamp recordings, which methodologically rule out potential effects of electric shunting, both amplitude and frequency of miniature inhibitory postsynaptic currents (mIPSCs) were unchanged across genotypes ( Supplementary Fig. 7a ). Unchanged mIPSCs also suggested that KCNQ5 had no effect on vesicle filling or release. Together, these experiments demonstrate that KCNQ5 contributes to the shunting of postsynaptic inhibitory activity. To examine the impact of KCNQ5 on synaptic transmission at the network level, we determined the input/output properties of the CA3 area in hippocampal slices. The slopes of field excitatory postsynaptic potentials (fEPSP), which reflect global postsynaptic responses of pyramidal cells upon stimulation of both glutamatergic and GABAergic inputs, were significantly smaller in Kcnq5 dn/dn than in WT mice ( Fig. 4k ). This difference was abolished in the presence of the GABA A receptor antagonist gabazine ( Fig. 4l ), demonstrating that the reduced postsynaptic response in Kcnq5 dn/dn mice was due to enhanced inhibition rather than decreased excitation of pyramidal cells. Hippocampal network oscillations and neuronal firing in vivo We next investigated how the changes in excitability and synaptic transmission as observed in brain slices translate into neuronal discharge and network oscillations in freely moving Kcnq5 dn/dn mice. The activity of putative pyramidal cells and interneurons was recorded using movable silicon probes and tetrodes in CA3 and CA1 areas during exploration, rest and sleep. The activity of Kcnq5 dn/dn CA3 pyramidal cells was changed as indicated by the reduced number of bursts ( Fig. 5a,b , Table 1 ). In line with our in vitro data demonstrating unaltered excitability of CA3 principal cells ( Supplementary Fig. 4b,c ), but increased excitability of CA3 interneurons ( Fig. 2 and Supplementary Fig. 4a ), overall average firing rates of CA3 pyramidal cells were not different between genotypes, whereas the average firing rates of fast-firing CA3 interneurons were significantly increased in Kcnq5 dn/dn mice ( Fig. 5b , Table 1 ). In contrast to unchanged average rates, the firing of Kcnq5 dn/dn CA3 pyramidal cells was reduced during gamma oscillations ( Fig. 5b and Table 1 ). 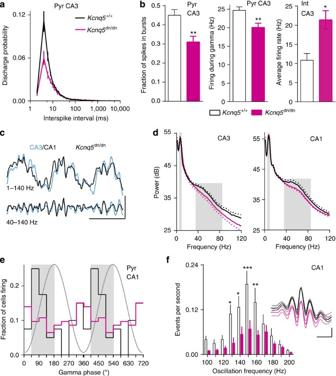Figure 5: Fast network oscillations inKcnq5dn/dnmicein vivo. (a) Interspike interval histograms demonstrating reduced CA3 pyramidal cell spiking at short intervals, that is, during bursts, inKcnq5dn/dnmice (mean±s.e.m.; WT: 39 cells, 4 mice,Kcnq5dn/dn: 22 cells, 4 mice). (b) Fraction of spikes emitted by pyramidal cells during bursts (left), discharge rate of CA3 pyramidal cells during gamma oscillations (middle), **P<0.01 (Student’st-test); firing rate of putative fast spiking interneurons (right; mean±s.e.m.; WT: 9 cells, 3 mice;Kcnq5dn/dn: 45 cells, 4 mice, *P<0.05, Wílcoxon rank sum test). (c) Gamma and concurrent theta oscillations in CA3 (blue) and CA1 (black) area. Example of LFP recording in a mutant mouse during running (wide-band and gamma band-pass filtered signals). Note covariance of gamma oscillation amplitude between the regions. Scale bars, 100 ms, 0.5 mV. (d) Power spectral density of the LFP from CA3 and CA1 during running (that is, during theta activity; CA3: WT andKcnq5dn/dn: 7 mice each; CA1, st. pyramidale: WT: 14 mice,Kcnq5dn/dn: 11 mice). Theta (5–10 Hz) and lower gamma (35–85 Hz) bands (grey shade). Power of gamma oscillations (integral power in the lower gamma band, CA3 and CA1 areas, and in the high gamma band, 85–120 Hz, CA3 area) is reduced inKcnq5dn/dnmice (P<0.05, Wilcoxon rank sum test). (e) Gamma phase preference of CA1 pyramidal cell firing. Mutants displayed reduced proportion of cells with preferred discharge phases between 45 and 180° (P<0.05, grey shade) and lower phase-locking (WT: 40 cells, 4 mice,Kcnq5dn/dn: 93 cells, 5 mice,P<0.05). Grey line—reference gamma oscillation cycle. (f) Reduced occurrence of slower (<170 Hz) ripple oscillations inKcnq5dn/dnmice (oscillatory events/s, mean±s.e.m., according to the event dominant frequency, WT: 10 mice,Kcnq5dn/dn: 11 mice), *P<0.05; **P<0.01; ***P<0.001 (Student’st-test). Inset: wide-band waveforms of ripples (mean±s.e.m.; WT: 10 mice,Kcnq5dn/dn: 11 mice). Scale bars, 10 ms, 0.1 mV. Figure 5: Fast network oscillations in Kcnq5 dn/dn mice in vivo . ( a ) Interspike interval histograms demonstrating reduced CA3 pyramidal cell spiking at short intervals, that is, during bursts, in Kcnq5 dn/dn mice (mean±s.e.m. ; WT: 39 cells, 4 mice, Kcnq5 dn/dn : 22 cells, 4 mice). ( b ) Fraction of spikes emitted by pyramidal cells during bursts (left), discharge rate of CA3 pyramidal cells during gamma oscillations (middle), ** P <0.01 (Student’s t -test); firing rate of putative fast spiking interneurons (right; mean±s.e.m. ; WT: 9 cells, 3 mice; Kcnq5 dn/dn : 45 cells, 4 mice, * P <0.05, Wílcoxon rank sum test). ( c ) Gamma and concurrent theta oscillations in CA3 (blue) and CA1 (black) area. Example of LFP recording in a mutant mouse during running (wide-band and gamma band-pass filtered signals). Note covariance of gamma oscillation amplitude between the regions. Scale bars, 100 ms, 0.5 mV. ( d ) Power spectral density of the LFP from CA3 and CA1 during running (that is, during theta activity; CA3: WT and Kcnq5 dn/dn : 7 mice each; CA1, st. pyramidale: WT: 14 mice, Kcnq5 dn/dn : 11 mice). Theta (5–10 Hz) and lower gamma (35–85 Hz) bands (grey shade). Power of gamma oscillations (integral power in the lower gamma band, CA3 and CA1 areas, and in the high gamma band, 85–120 Hz, CA3 area) is reduced in Kcnq5 dn/dn mice ( P <0.05, Wilcoxon rank sum test). ( e ) Gamma phase preference of CA1 pyramidal cell firing. Mutants displayed reduced proportion of cells with preferred discharge phases between 45 and 180° ( P <0.05, grey shade) and lower phase-locking (WT: 40 cells, 4 mice, Kcnq5 dn/dn : 93 cells, 5 mice, P <0.05). Grey line—reference gamma oscillation cycle. ( f ) Reduced occurrence of slower (<170 Hz) ripple oscillations in Kcnq5 dn/dn mice (oscillatory events/s, mean±s.e.m., according to the event dominant frequency, WT: 10 mice, Kcnq5 dn/dn : 11 mice), * P <0.05; ** P <0.01; *** P <0.001 (Student’s t -test). Inset: wide-band waveforms of ripples (mean±s.e.m. ; WT: 10 mice, Kcnq5 dn/dn : 11 mice). Scale bars, 10 ms, 0.1 mV. Full size image Table 1 Neuronal excitability in vivo . Full size table Network oscillations coordinate the activity of neuronal populations and are believed to be crucial for cognitive processes [34] . They occur in different frequency ranges and can be recorded as changes in the extracellular local field potential (LFP). Gamma frequency band (35–85 Hz) oscillations of area CA3 shape gamma oscillations in the CA1 region in rats [35] . We now found a similar synchronization between CA3 and CA1 LFP in mice ( Fig. 5c ). In Kcnq5 dn/dn mice, the power of gamma oscillations (35–85 Hz) was decreased in both CA3 and CA1 areas ( Fig. 5d and Supplementary Table 1 ) and the distribution of the preferred discharge phases of individual pyramidal cells was altered ( Fig. 5e ). Whereas in control mice ~42% of neurons preferentially fired during the ascending phase of the gamma cycle (‘RisPyr’ cells [36] ), in Kcnq5 dn/dn mice only ~25% of cells fired preferentially during this phase ( Fig. 5e ). During theta oscillations, WT pyramidal cells showed a strong preference for the depolarizing part of the theta cycle during which CA3 area-generated gamma oscillations [37] and the maximal discharge of RisPyr [36] are typically observed. In contrast, the discharge of Kcnq5 dn/dn pyramidal cells was more uniformly distributed along the theta cycle ( Supplementary Fig. 8a ). Theta oscillations (5–10 Hz) did not differ between genotypes ( Fig. 5d and Supplementary Table 1 ). The CA3 and CA1 networks also participate in the synchronization underlying high-frequency oscillations (140–200 Hz, ‘ripples’) in CA1 during rest and sleep [38] , [39] . Whereas the power spectra of ripples were similar in WT and Kcnq5 dn/dn mice ( Supplementary Fig. 8b and Supplementary Table 1 ), their occurrence was markedly reduced in mutants ( Fig. 5f ). Thus, fast network oscillations were attenuated in Kcnq5 dn/dn mice, whereas synchronization at lower frequencies (theta, 5–10 Hz) remained intact. Changes in spatial representations in Kcnq5 dn/dn mice In freely moving mice, CA1 pyramidal cells displayed no significant changes of average firing rates, number of spikes per burst or intraburst discharge frequency between the genotypes ( Table 1 ). However, Kcnq5 dn/dn CA1 pyramidal cells fired more bursts ( Table 1 ), consistent with the apparent reduction of RisPyr cells, which display lower burst probability [36] . Firing of CA1 pyramidal cells as a function of the spatial position of the mouse was analyzed during exploration of a circular arena. Peak firing rate and spatial coherence of pyramidal cells’ activity were largely similar between genotypes ( Fig. 6a,b and Supplementary Table 2 ). However, Kcnq5 dn/dn mice displayed larger place field sizes and increased firing rates averaged over the entire arena ( Fig. 6b and Supplementary Table 2 ). Thus, our results indicate unaltered overall excitability but impaired spatial representations in the CA1 area in Kcnq5 dn/dn mice. By contrast, spatial firing of CA3 pyramidal cells did not differ between genotypes except for reduced peak firing rates in the mutant ( Supplementary Fig. 9 ). 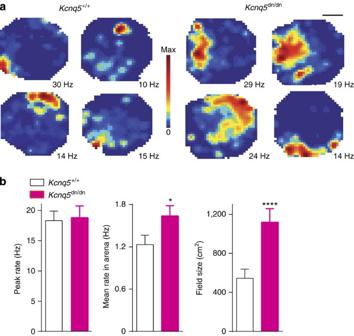Figure 6: Spatial representations in the CA1 area ofKcnq5dn/dnmice. (a) Firing maps of CA1 pyramidal cells recorded in a circular arena. The spiking activity of single place cells at each particular location is colour-coded (linear scale from zero to max shown in center). It is normalized to the peak firing rate of respective place cells, which is given as number in the right lower corner of each map. Scale bar (top right), 0.2 m. (b) Spatial firing properties of CA1 pyramidal cells recorded during exploration in the arena: peak rate (highest firing rate across all spatial bins), mean rate (over all spatial bins) and place field size (mean±s.e.m.; WT: 37 cells, 4 mice;Kcnq5dn/dn: 36 cells, 4 mice), *P<0.05; ****P<0.0001 (Wilcoxon rank sum test). Figure 6: Spatial representations in the CA1 area of Kcnq5 dn/dn mice. ( a ) Firing maps of CA1 pyramidal cells recorded in a circular arena. The spiking activity of single place cells at each particular location is colour-coded (linear scale from zero to max shown in center). It is normalized to the peak firing rate of respective place cells, which is given as number in the right lower corner of each map. Scale bar (top right), 0.2 m. ( b ) Spatial firing properties of CA1 pyramidal cells recorded during exploration in the arena: peak rate (highest firing rate across all spatial bins), mean rate (over all spatial bins) and place field size (mean±s.e.m. ; WT: 37 cells, 4 mice; Kcnq5 dn/dn : 36 cells, 4 mice), * P <0.05; **** P <0.0001 (Wilcoxon rank sum test). Full size image We have used a genetic mouse model expressing a non-conducting dominant negative, trafficking-impaired KCNQ5 mutant to disrupt the function of KCNQ5-containing K + channels in the brain and to investigate its physiological role using electrophysiological techniques both in vivo and in vitro . We found that KCNQ5 is an important modulator of synaptic inhibition in the CA3 area. Loss of KCNQ5 function changed fast network oscillations and modified spatial discharge of pyramidal cells in freely moving mice. Constitutive gene disruption may entail secondary changes that can sometimes be compensatory. We cannot exclude that the loss of KCNQ5 channel function, or even the mislocalization of the nonfunctional protein, may have changed the expression of some genes in Kcnq5 dn/dn mice or may have had other secondary effects. However, the expression of KCNQ2 and KCNQ3 was unchanged in Kcnq5 dn/dn brain [13] , and here we found neither changes in Kcnq5 mRNA levels, nor in those of several Kir K + channels. Moreover, the levels of several synaptic proteins were unaltered in Kcnq5 dn/dn brain and no change in CNS morphology could be detected. Importantly, our ‘dominant-negative’ strategy, in which all heteromeric channels containing one or more KCNQ5 subunit(s) are inactivated, avoided the possibility of the formation of more efficient KCNQ2/3 heteromers that may occur in Kcnq5 −/− mice. KCNQ2, -3 and -5 are broadly expressed in the brain and show robust expression in the hippocampus [13] , [19] , [32] , [33] . All three isoforms, as well as KCNQ2/3 and KCNQ3/5 heteromers, mediate K + currents that slowly activate upon membrane depolarization. These channels are ideally suited to control neuronal excitability because they are partially open at resting voltages and can be inhibited by various G-protein-coupled receptors. Despite these similarities, KCNQ isoforms have different physiological roles, as illustrated by epilepsy which was described for mutations in KCNQ2 or KCNQ3 , but not KCNQ5 (ref. 40 ). Whereas slightly different biophysical properties may play a role in determining the divergent roles of KCNQ isoforms, differences in expression patterns may have a larger impact. KCNQ2 and -3 are robustly expressed in CA1 pyramidal cells and granule cells [41] , whereas KCNQ5 shows higher expression in the CA3 area [13] where we demonstrated its localization in pyramidal cells and interneurons. Even more important may be the divergent subcellular localization. KCNQ2/KCNQ3 channels are targeted to axon initial segments and nodes of Ranvier, structures involved in action potential generation and conduction, respectively. Neither subunit was detected at hippocampal synapses [32] . The localization of KCNQ2 and -3 at axon initial segments of excitatory neurons agrees excellently with their role in epilepsy. By contrast, we could not detect KCNQ5 at axon initial segments, but rather observed intense KCNQ5-positive puncta at inhibitory synapses in several brain regions. The relocation of the trafficking-deficient KCNQ5 mutant to pyramidal cell bodies, together with subcellular fractionation and STED microscopy strongly suggested a postsynaptic localization of WT KCNQ5 on pyramidal cells. Others have described KCNQ5 in the presynaptic calyx of Held [22] , [23] . However, we found that KCNQ5 did not co-localize with markers for excitatory synapses at the presynaptic membrane of this giant synaptic terminal, but rather with gephyrin, a postsynaptic protein of inhibitory synapses, at the outer face of the calyx that directly receives inhibitory input [31] . However, KCNQ5 is also found in the postsynaptic membrane of vestibular calyx synapses [24] that receives excitatory input from ensheathed vestibular hair cells. Hence, in principle, KCNQ5 might be expressed in postsynaptic membranes of both inhibitory and excitatory synapses. We cannot rule out that excitatory synapses in the hippocampus express KCNQ5 at levels that are below the detection threshold of our labelling technique. Likewise, the sensitivity of our antibody may not be high enough to detect the protein when it is uniformly distributed over neuronal plasma membranes. Unambiguous detection of KCNQ5 in interneurons was only possible in Kcnq5 dn/dn mice in which the mutant protein accumulated in cell bodies. We suspect that KCNQ5 expression in interneurons is not limited to the rather small subset of cells identified by robust KCNQ5 accumulation because this fraction seems too small to account for the general increase in CA3 interneuron excitability in Kcnq5 dn/dn mice. KCNQ5 dampens synaptic inhibition at both main cellular sites of expression in CA3, that is, at interneurons and pyramidal cells. Interneurons lacking functional KCNQ5 were hyperexcitable as evident from current injection experiments and from increased frequency of spontaneous IPSCs of their target cells. This hyperexcitability is most likely a direct, cell-autonomous effect of the loss of a KCNQ5-mediated plasma membrane conductance since excitability was assessed in the absence of synaptic transmission. This increase in excitability, which was found for all classes of interneurons investigated here, is consistent with the role of KCNQ channels in stabilizing the membrane potential and in spike-frequency adaptation [15] . Although KCNQ5 may additionally dampen synaptic inhibition by shunting inhibitory postsynaptic currents, our findings suggest that the increased excitability of interneurons is the predominant mechanism that increases inhibition in our mouse model. Ambient GABA is predominantly derived from synaptic vesicles released by interneurons [42] , which are more excitable in Kcnq5 dn/dn mice. Indeed, tonic GABA currents, which have been described previously in the CA3 region [43] , were enhanced in our mutant mice, suggesting that both tonic and phasic GABA contributes to the overall increase in inhibition in Kcnq5 dn/dn mice. Importantly, modulation of KCNQ5 activity appears to be physiologically relevant as muscarinic stimulation increased the frequency of spontaneous IPSCs in WT, but not in Kcnq5 dn/dn slices. Unlike interneurons, pyramidal cells of Kcnq5 dn/dn mice showed no increased excitability, suggesting that KCNQ5, in contrast to KCNQ2/3 in CA1 neurons [17] , contributes little to the K + conductance at the spike initiation zone or that the excitability of CA3 pyramidal cells is under homeostatic control. Importantly, increased firing rates of Kcnq5 dn/dn CA3 interneurons, but not of pyramidal cells, were also observed in vivo . The activity of large neuronal populations is organized by hippocampal network oscillations, which are thought to be crucial for cognitive processes [34] , [37] , [44] . Loss of KCNQ5 function selectively impaired gamma (35–85 Hz) and ripple (140–200 Hz) oscillations without affecting slower oscillations in the theta band (5–10 Hz), a finding differing from those of mouse models targeting other proteins involved in hippocampal excitability [45] , [46] , [47] , [48] . During 35–85 Hz gamma oscillations CA1 networks follow the rhythm generated in the CA3 area [35] . Therefore, the changes in CA1 gamma oscillations of Kcnq5 dn/dn mice likely result from changed synchronization in the CA3 area, where KCNQ5 expression is higher (see ref. 13 and present work). Network oscillations emerge from the coordinated interaction of neuronal excitation and inhibition [49] , [50] . In computational models, excitatory cells drive the activity of interneurons resulting in delayed feedback inhibition. Modulation of this inhibitory feedback, as well as the magnitude and temporal pattern of the excitatory drive, are key factors in shaping gamma oscillations [49] . These aspects of excitability directly depend on network inhibition, which is modified in Kcnq5 dn/dn mice. Furthermore, reduced AHP currents in the CA3 pyramidal cells in Kcnq5 dn/dn mice [13] might have also contributed to impairment of gamma-rhythmic firing [51] . Less irregular spiking of CA3 pyramidal cells (reduced burst firing, as observed here) counteracts gamma synchronization in a computational model [49] , in line with reduced gamma oscillations in Kcnq5 dn/dn mice. Optogenetic silencing of interneurons increases CA1 pyramidal cell burst firing in vivo [52] . Conversely, the increased excitability of CA3 interneurons might lead to decreased burst firing of Kcnq5 dn/dn CA3 pyramidal cells. Increased inhibition in the CA3 area could also be a cause of the reduced occurrence of otherwise intact ripple oscillations in the Kcnq5 dn/dn CA1 area. Collective discharge of large neuronal populations in the CA3 area, so called sharp-wave bursts, provide excitatory drive required for generation of ripples in the CA1 area [39] (but see ref. 53 ). Increased inhibition in the CA3 of Kcnq5 dn/dn mice could lead to less frequent generation of sharp-waves, which, like other forms of population bursts in the CA3 area, rely on the excitability of the CA3 network [39] , [54] . Hence, both decreased gamma and ripple oscillations as well as decreased burst firing of CA3 pyramidal cells and reduced peak firing rates in CA3 place fields in Kcnq5 dn/dn mice likely arise from increased synaptic inhibition in the CA3 area. Signalling from CA3 to CA1 area during gamma oscillations is believed to influence positional firing of pyramidal cells [36] , [55] . Chemical ablation of the CA3 area [56] or its functional genetic disconnection from the CA1 area [57] lead to less sharp [56] and enlarged [57] CA1 place fields. Kcnq5 dn/dn mice display enlarged CA1 place fields suggesting that gamma-frequency synchronization in the CA3 and CA1 areas may be crucial for precise spatial coding in CA1. In line with our results, enlarged place fields accompanied by memory deficits were observed after blocking the CA3 output [57] . Although our present in vitro findings point out functions of hippocampal KCNQ5 channels, other brain regions, which also express KCNQ5, might to some extent also contribute to the observed change in place fields. Although it seems likely that KCNQ5 dampens excitation not only in hippocampus, but also in other brain regions, such a generalization will require experimental verification. Using a genetic approach we identified specific roles of KCNQ5 that set this isoform apart from KCNQ2 and -3, both of which are also widely expressed in brain. A major difference between these KCNQ isoforms is their global role in network excitability. Both KCNQ2 and - 3 are mutated in human neonatal epilepsy [3] , [4] , [58] , and mouse models with reduced KCNQ2 or KCNQ3 function display reduced seizure thresholds, epileptic discharges or overt epilepsy [17] , [59] , [60] . By contrast, Kcnq5 dn/dn mice neither displayed seizures [13] nor epileptic discharges in vivo . This difference may be explained by differences in expression patterns. Loss of KCNQ2/3 function increases network excitability because these channels are prominently localized at spike initiation zones of excitatory neurons, whereas loss of KCNQ5 rather dampens hippocampal excitability because it is expressed in interneurons and at inhibitory synapses. As a consequence, Kcnq5 dn/dn mice did not exhibit the strong neurological phenotype observed in KCNQ2/3 mouse models. Animals Kcnq5 dn/dn mice [13] and GAD67-GFP mice [26] have been described previously and were studied in a C57BL/6 genetic background. Mice were housed under standard conditions in the animal facility of the MDC according to institutional guidelines and kept on a 12-h light/dark cycle. For all experiments, age-matched mice, preferably littermates, were used. All procedures were performed in accordance with national and international guidelines and were approved by the local health authority (Landesamt für Gesundheit und Soziales (LaGeSo), Berlin). Males between age 4 and 25 weeks were used. All mice were kept in their home cages for 3 days to acclimate before testing. Antibodies The following antibodies were used for immunohistochemistry: rabbit anti-KCNQ5, rabbit anti-KCNQ3, rabbit anti-KCNQ2 (see ref. 13 ; 1:200–1:500); mouse anti-gephyrin (Synaptic Systems m7Ab; 1:200); mouse anti-Ankyrin G (Zymed; 1:50); mouse anti-vGAT (Synaptic Systems; 1:300); guinea pig anti-vGlut1 (Millipore, 1:1,000); mouse anti-GluR2 (Millipore, 1:500); mouse anti-GAD65/67 (Biotrend, 1:2,000); mouse anti-bassoon (Abcam, 1:400); mouse anti-calbindin (Sigma, 1:2,000); goat anti-GluRδ2 (Santa Cruz, 1:200); guinea pig anti-parvalbumin (Synaptic Systems, cat.# 195004, 1:200); goat anti-calretinin (Millipore cat.# AB1550, 1:500); goat anti-somatostatin (Santa Cruz, cat.# 7819, 1:200); rabbit anti-NPY (Abcam, cat.# ab30914, 1:1,000); chicken-anti GFP (Aves, 1:500). Secondary antibodies were Alexa Fluor 555 goat anti-rabbit IgG; Alexa Fluor 488, goat anti-mouse IgG; Alexa Fluor 488, goat anti-guinea pig IgG; Alexa Fluor 488 donkey anti-goat IgG (Molecular Probes). Secondary antibodies for STED microscopy were goat anti-rabbit IgG Atto 647N (Sigma; 1:200) and goat anti-mouse IgG Chromeo 494 (Active Motif, Carlsbad, USA, 1:50) or goat anti-mouse Abberior Star 580 (Abberior Göttingen, Germany). For diaminobenzidine (DAB) peroxidase labelling HRP-conjugated secondary antibodies were used (DAKO Envision+HRP system). For co-staining KCNQ5 with NPY ( Supplementary Fig. 2C ), we used a new anti-KCNQ5 antibody that had been raised in guinea pigs against the carboxyterminal peptide CKTGDSTDALSLPHVKLN (coupled to KLH). After purification against the peptide, it proved to be specific in western blots and immunohistochemistry. Immunohistochemistry Immunohistochemistry was performed on paraffin sections as described previously [13] . Nuclei were stained with 4′,6-diamidino-2-phenylindole (DAPI). Sections were imaged using a Zeiss LSM 510 confocal microscope. Image analysis was performed off-line with ZEN 2009 light edition software (Zeiss) and Adobe Photoshop (Adobe Systems). DAB-stained sections were examined with a Zeiss Axiophot or Zeiss Stemi-2000-c microscope. For quantification of DAB stainings of Kcnq5 +/+ and Kcnq5 dn/dn hippocampus, the ImageJ 1.36b elliptic selection function was used and the region of interest (2,166 pixels) was either marked in CA3 st. oriens, st. pyramidale or st. radiatum close to CA1/CA2 region and DAB signal intensities were measured. The DAB signal ratios=[st. oriens/st. pyramidale] or [st. radiatum/st. pyramidale] were calculated for individual mice and compared using Student’s paired two-tailed t -test. For all quantifications, sections from at least three animals/genotype were analyzed. STED microscopy For distance measurements between KCNQ5 and bassoon, gephyrin and homer, respectively, immune-labelled paraffin sections (8 μm) were mounted in 2′,2′-thiodieethanol (TDE). The sections were immersed with increasing TDE concentrations in PBS buffer (10, 25, 50, 97%, 10 min each) and finally embedded in 97% TDE. STED imaging was performed by using a commercial two-channel STED microscope (Leica Microsystems) as described previously [61] . Briefly, the system consists of an inverted microscope (DMI 6000 CS with a Tandem Scanning System SP5) equipped with two pulsed excitation lasers of 532 and 635 nm (≈70 ps pulse width, 80 MHz repetition rate; PicoQuant) and a Titanium saphire laser (Chameleon ultra II (≈100 fs pulse width, 80 MHz repetition rate), Coherent) as depletion light source. STED-stacks, consisting of at least six slices were acquired sequentially with a × 100HCX PL APO CS oil objective (Leica Microsystems). STED-depletion was done at 730 nm (Abberior-dye) and at 750 nm (Atto-dye) Scanning-format of 1,024 × 1,024 and zoom of six resulted in a pixel size of 25, 2 nm ( x , y ) and 126 nm ( z ). Scan speed was set to 700 Hz with line averaging of 48. Fluorescence signals were detected sequentially by avalanche photo diodes (Perkin Elmer Inc.) within two spectral regions (589–625 nm for Abberior STAR 580) and 655–685 nm for Atto 647N) separated by a dichroic beam splitter at 650 nm. To enhance focus stability and minimize thermal drift, the microscope was housed in a light tight customized heatable incubation chamber (Pecon). Following image acquisition, the raw data were deconvolved using Huygens Professional 4.4 (Scientific Volume Imaging B.V) software. Deconvolution was done by using the pulsed STED optimized function to calculate a theoretical point spread function out of the specific microscope parameter. Default deconvolution parameters were applied. To measure the distances between KCNQ5 and Bassoon, Gephyrin or Homer, respectively, slices from the centre of the stack were chosen by using the Huygens Twin Slicer. A line profile plot from peak to peak was created manually and distance values registered. Subsequent statistical analysis was done with GraphPad Prism 5 (GraphPad Software, Inc.). Further image processing was done by using ImageJ (National Institutes of Health) and Photoshop CS 5 (Adobe System Inc.). Tissue preparation for electrophysiology Mice of age 4–6 weeks were deeply anaesthetized with isoflurane, killed by decapitation and brains were removed. Horizontal hippocampal slices (400 μm) were cut using a Leica VT1200S vibratome. Different preparation solutions were used. For all recordings, the tissue was prepared in ice-cold, saccharose-based artificial cerebrospinal fluid (ACSF) (in mM): NaCl 87, Na 2 PO 4 1.1, NaHCO 3 28.8, KCl 2.5, CaCl 2 0.5, MgSO 4 7, saccharose 75 and glucose 11 at a pH of 7.4 gassed with carbogen. Slices were kept in saccharose-based ACSF at 34.5 °C for ~30 min and subsequently maintained in physiological ACSF (in mM): NaCl 129, Na 2 PO 4 1.1, NaHCO 3 28.8, KCl 2.8, CaCl 2 2.5, MgSO 4 1.3 and glucose 10 at a pH of 7.4 at room temperature. All subsequent in vitro recordings were performed at a temperature of 32–34 °C. Field potential recordings Recording and stimulation electrodes (2–4 MΩ) were filled with ASCF and placed in the st. radiatum of the CA3 area. fEPSPs were evoked at 0.1 Hz. Only experiments with clearly detectable fibre volleys were used for analysis. During input–output measurements, the stimulus strength was adjusted and at least three independent measurements for every stimulation step were performed in order to achieve the desired fibre volley amplitudes. To minimize the error caused by potential population spike contamination in all experiments, we analyzed the slope of the fEPSP instead of the fEPSP amplitude. Furthermore, all traces with unusual time course of the initial slope were excluded from analysis. Patch-clamp recordings Recordings were performed in the whole-cell configuration. Hippocampal pyramidal neurons (CA3/CA1) were identified with differential interference contrast microscopy. Interneurons were identified by GFP fluorescence in mice expressing the GAD67-GFP allele [26] in a heterozygous state. Recordings were performed in interneurons from st. oriens, st. pyramidale and st. radiatum. In recordings from st. oriens and st. pyramidale, interneurons were filled with biocytin (0.3–0.5%) to allow post-hoc anatomical reconstruction of axonal arborization and subsequent classification into oriens-lacunosum-moleculare cells, bistratified cells and basket cells (see below). Interneurons from st. radiatum were not filled with biocytin and pooled into one group for analysis. Pipettes were pulled from borosilicate glass (Hilgenberg). Pipette resistances were ~4–6 MΩ. Patch-clamp recordings were performed with MultiClamp 700B, a Digidata 1,440 A interface and PClamp software (Molecular Devices). Signals were low-pass filtered at 3 kHz and digitized at 10 kHz. Recordings with series resistance >30 MΩ were discarded. Action potentials were recorded in current clamp mode using a K-methylsulphonate-based pipette solution (in mM): 130 K-methylsulphonate, 4 KCl, 4 NaCl, 4 MgATP, 0.3 Na 2 GTP, 0.2 EGTA, 10 phosphocreatine and 10 HEPES. ACSF was supplemented with 1 μM gabazine, 50 μM D (-)-2-amino-5-phosphonovaleric acid (AP5) and 10 μM 6-cyano-7-nitroquinoxaline-2,3-dione (CNQX). Membrane potential values were not corrected for liquid junction potentials. Cells with resting membrane potential above −50 mV were discarded. Evoked and spontaneous postsynaptic currents (sIPSCs including ambient GABA recordings, mIPSCs sEPSCs and evoked IPSCs (eIPSCs)) were recorded in voltage clamp mode at −70 mV holding potential using a high chloride internal solution containing (in mM): 130 CsCl, 2 MgCl 2 , 2 MgATP, 10 HEPES, 0.2 EGTA and 5 QX-314, pH 7.2 (290 mOsm l −1 ). sIPSCs and mIPSCs were recorded in ASCF supplemented with CNQX (10 μM) and AP5 to block α-amino-3-hydroxy-5-methyl-4-isoxazole propionic acid and N -methyl- D -aspartate receptors, respectively. For mIPSC recordings, ACSF was additionally supplemented with 1 μM tetrodotoxin (TTX). sEPSCs were measured in the presence of 1 μM gabazine to block GABA-A receptors. For eIPSCs, stimulation was performed with an ACSF-filled patch pipette [62] placed in st. radiatum of the CA3 area (<0.2 mm from the tip of the recording electrode). eIPSCs were recorded in the presence of CNQX and AP5. Miniature postsynaptic potentials (mIPSPs) were recorded in current clamp mode at a voltage between −60 and −65 mV (or −85 and −90 mV) using a KCl-based pipette solution (in mM): 135 KCl, 2 MgCl 2 , 2 MgATP, 0.2 EGTA and 10 HEPES (290 mosm, pH 7.2). ACSF was supplemented with 1 μM TTX, 50 μM AP5 and 10 μM CNQX. Cells with resting potential more positive than −50 mV were discarded. The following bath-applied drugs were used: AP5 50 μM, CNQX 10 μM, TTX 1 μM, QX314, SR95531 (gabazine) 1 or 10 μM (ambient GABA recordings), carbachol 20 μM. Drugs were purchased from Tocris or Sigma-Aldrich. Statistical analysis of in vitro data Unless otherwise stated, Student’s t -test (paired and non-paired) or analysis of variance (SPSS) were used where appropriate. Statistical significance level was set to P <0.05 and marked in figures by asterisks (*). All data were analyzed using Clampfit (Molecular Devices), Prism (GraphPad Software) and Matlab (MathWorks). Spontaneous events were analyzed with MiniAnalysis (SynaptoSoft Inc.) using a threshold-based search paradigm and visual post hoc inspection. Histograms of synaptic events were derived from at least 200 events per cell. Slice processing and reconstruction of biocytin-filled cells For anatomical reconstruction, cells were loaded with 0.3–0.5% biocytin. After finished recordings, slices were transferred to 4% paraformaldehyde for overnight fixation and were then maintained in 0.1 M phosphate buffer. For histological processing, the slices were re-sectioned (100 μm). Biocytin-filled cells were subsequently visualized with 3,3′-diaminobenzidine tetrahydrochloride (0.015%) using a standard ABC kit (Vectorlabs, Burlingame, CA, USA) and reconstructed on a light microscope at × 40 or × 60 with a Neurolucida 3D reconstruction system (MicroBrightField). In vivo electrophysiology Kcnq5 dn/dn and control mice were implanted in the dorsal hippocampus with microdrives (Minidrive-8, BioSignal Group) loaded with tetrodes (independently movable, fabricated from a 12-μm tungsten wire, California Fine Wire Company, 4 mice), 32-site (4 octrodes/probe) silicon probes (B32, Neuronexus Technologies, 9 mice) or arrays of single tungsten wires (40 μm, California Fine Wire Company, 6 mice) mounted on custom microdrives as well as with linear silicon probes (CM32, Neuronexus Technologies, 13 mice) or with not movable arrays of tungsten wires (12 mice). Electrodes were implanted under isoflurane anaesthesia above the hippocampus and subsequently positioned in the CA1 or CA3 pyramidal cell layer, using LFP and unitary activity as a reference. Reference and ground electrodes were miniature stainless-steel screws in the skull. Implanted electrodes and microdrive were secured on the skull with dental acrylic. Recordings were performed during exploration in a round arena (60 cm in diameter) for 10–15 min as well as during awake immobility and sleep in the home cage. A light-emitting diode was attached to the headset to track the animal’s position during exploration. Electrodes were connected to operational amplifiers (Noted B.T.) to eliminate cable movement artefacts. Electrophysiological signals were differentially amplified, band-pass filtered (1 Hz–10 kHz, Digital Lynx) and acquired continuously at 32 kHz. After completion of the experiments, mice were deeply anaesthetized and electrolytic lesions at selected recording sites were performed. Subsequently, the animals were perfused intracardially with 4% paraformaldehyde solution and decapitated. Brains were fixed, cut in 40 μm slices, stained with cresyl violet and recording sites were confirmed. Signal processing was carried out off-line by custom-written MATLAB (Mathworks) and occasionally by C algorithms [46] , [48] , [63] . LFP was processed by low-pass filtering and down-sampling of the wide-band signal to 1,250 Hz. Recordings from st. pyramidale used for further analyses were selected as described previously [48] . Theta oscillations were detected automatically in the recordings during running based on theta/delta power ratio of at least 6. Power spectral density was computed using the multitaper method ([NW]=3, window size 1,024). For group comparisons, power spectra were standardized to the power in the delta (1–4 Hz) band. Cumulative power was computed as a sum of power in a given frequency band. Ripple oscillations were detected as described previously [63] . Action potentials were detected in a band-pass filtered signal (0.8 Hz–5 kHz). Events with a magnitude exceeding 3 s.d. above mean were detected, spike waveforms were extracted and represented by the first three principle components. Spike sorting was performed automatically [64] followed by manual clusters adjustment [65] . Putative pyramidal cells and interneurons were identified based on their autocorrelograms and firing rate (<3 Hz for pyramidal cells, >7 Hz for putative basket cells). Single pyramidal cells with a clear refractory period (>2 ms) as well as single and multiunit-interneurons were used in further analysis. Bursts were defined as a series of spikes separated by intervals of no more than 15 ms. Intraburst discharge frequency was computed as a burst duration divided by the number of interspike intervals in a burst. The oscillation phase was extracted by linear interpolation between wave peaks and troughs in respective frequency bands during detected oscillation epochs. Mean phase and the resultant vector length were computed for each individual spike train. Firing maps of pyramidal cells were computed by dividing the number of spikes in a given spatial pixel (2 × 2 cm) by the time spent in this pixel. Periods of immobility were excluded from the analysis. Peak firing rate was defined as the maximum firing rate over all pixels in the environment. Coherence, a measure of the local smoothness of the firing profile, was computed as the Fisher z-transform of the Pearson’s correlation between the rate in a given pixel and the average rate in its eight first-order neighbours. Place fields were detected as spatially continuous areas where the firing rate exceeded 1 Hz. Mean firing rate across all pixels of a place field and the place field size were computed for the largest place field in a session. The statistical significance of single comparisons was determined by the Wilcoxon’s rank sum test or with t -test depending on the distribution normality (determined by the Lilliefors test) as well as by the χ 2 test for comparisons of proportions. Circular statistics was performed using Rayleigh and Watson-Williams tests. How to cite this article: Fidzinski, P. et al . KCNQ5 K + channels control hippocampal synaptic inhibition and fast network oscillations. Nat. Commun. 6:6254 doi: 10.1038/ncomms7254 (2015).